Densified network glasses and liquids with thermodynamically reversible and structurally adaptive behaviour If crystallization can be avoided during cooling, a liquid will display a substantial increase of its viscosity, and will form a glass that behaves as a solid with a relaxation time that grows exponentially with decreasing temperature. Given this ‘off-equilibrium’ nature, a hysteresis loop appears when a cooling/heating cycle is performed across the glass transition. Here we report on molecular dynamics simulations of densified glass-forming liquids that follow this kind of cycle. Over a finite pressure interval, minuscule thermal changes are found, revealing glasses of ‘thermally reversible’ character with optimal volumetric or enthalpic recovery. By analysing the topology of the atomic network structure, we find that corresponding liquids adapt under the pressure-induced increasing stress by experiencing larger bond-angle excursions. The analysis of the dynamic behaviour reveals that the structural relaxation time is substantially reduced in these adaptive liquids, and also drives the reversible character of the glass transition. Ultimately, the results substantiate the notion of stress-free (Maxwell isostatic) rigidity in disordered molecular systems, while also revealing new implications for the topological engineering of complex materials. Certain materials, when cooled fast enough through their melting point, can remain in a metastable supercooled state and, upon further cooling, can eventually freeze into a glass at a reference temperature T g , which is usually associated [1] , [2] with a viscosity of 10 12 Pa s or a relaxation time of 100 s. As the temperature of the liquid is lowered, viscosity and the relaxation time towards thermodynamic equilibrium will increase markedly. However, even in the obtained glassy state, the material will continue to relax to a lower energy state but on timescales that exceed the laboratory timescale by several orders of magnitude. To track such subtle effects, one conventionally uses calorimetry to measure the heat capacity of the glass and the liquid, and with heating a hysteresis loop appears [3] , [4] , causing a heat capacity overshoot at the glass transition. This endotherm peak simply reveals that previously frozen degrees of freedom during the quench are now excited, so that the overshoot is a direct manifestation of the relaxation taking place between room temperature and T g . Here we show by using molecular dynamics (MD) simulations that for a fixed cooling/heating rate this hysteresis can be minuscule under certain thermodynamic conditions, and defines a calorimetric reversibility window (RW) and a volume recovery window, while also underscoring an obvious anomalous relaxation behaviour that is characterized. A direct connection is made with the softening of bond angles at the molecular level, which adapt under the pressure-driven increasing stress leading to a growth of the atomic coordination numbers, and network connectivity. It is found that such ‘thermally reversible’ glasses are stress-free, and bear striking similarities with calorimetric anomalies in modified glassy alloys, while also satisfying the well-known Maxwell stability criterion of isostatic mechanical structures [5] , [6] , and displaying anomalous relaxation dynamics in the supercooled regime. These findings open the possibility to use stress-free rigidity for the design of a variety of functionalities in disordered materials, an original perspective that is directly derived from basic findings, and which has inspired the recent development of topological engineering of commercial glasses. Glass transition cycle To establish our conclusions, we use as a target system a densified sodium silicate liquid (2SiO 2 –Na 2 O or NS2) that is investigated by MD in ( N , V , T ) and ( N , P , T ) ensembles (see Methods Summary in refs 7 , 8 , 9 ). These materials are made of SiO 4/2 tetrahedra that are connected by bridging oxygens (BOs) whereas sodium cations create in their immediate vicinity so-called non-BOs (NBO), which contribute to the depolymerization of the network structure ( Fig. 1 ) [10] . 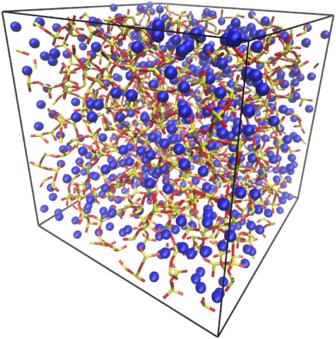Figure 1: Structure of a densified silicate. Snapshot of a sodium disilicate (2SiO2–Na2O, NS2) glass at room temperature. The structure is composed of network-forming species Si (yellow) and O (red), and cations (Na, blue spheres). Figure 1: Structure of a densified silicate. Snapshot of a sodium disilicate (2SiO 2 –Na 2 O, NS2) glass at room temperature. The structure is composed of network-forming species Si (yellow) and O (red), and cations (Na, blue spheres). Full size image We systematically perform isobaric/isochoric cycles, and start from an equilibrated liquid configuration at 3,000 K, and then cool the system at a rate of 1 K ps −1 to 300 K. The simulations reproduce the phenomenology of the glass transition temperature ( Fig. 2 , and Methods), that is, a slower cooling (from 10 to 0.1 K ps −1 ) leads to lower glass energies and a fictive temperature (the temperature at which the system deviates from its equilibrium line) that is lower. The crossover between the low-temperature and high-temperature linear expansion permits one to determine a fictive temperature, in very much the same fashion as in experiments. Once in the glassy state, we subsequently anneal the system back to the initial temperature at the same rate. The same procedure is then repeated at different pressures/volumes. Figure 3a shows the behaviour of the volume for selected pressures (0, 8 and 16 GPa) during the MD cycle (see also Fig. 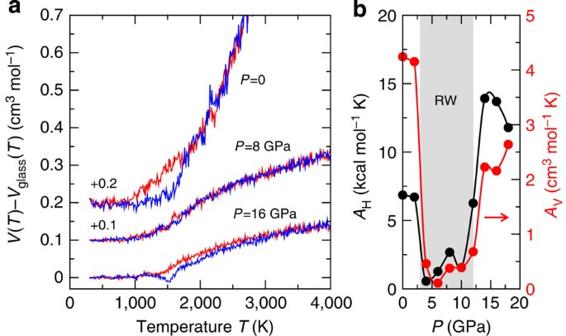Figure 3: Effect of pressure on the cooling/heating cycle across the glass transition. (a) Volume-temperature dependence in (N,P,T) ensemble during a cooling (red) and heating (blue) cycle for selected pressures of liquid 2SiO2–Na2O across the glass transition. The volumes have been rescaled with respect to their evolution in the glassy stateVglass(T). Curves at 0 and 8 GPa have been shifted by multiples of 0.1. The cycle leads to a hysteresis, which is due to structural relaxation. (b) Area of the enthalpic (AH) and volumetric (AV, red curve, right axis) hysteresis as a function of the applied pressureP, defining a reversibility window (RW, grey zone). 2b ). Because of the off-equilibrium nature of glasses, one usually obtains a hysteretic behaviour for volume or enthalpy driven by the relaxation, and this is, in fact, recovered in the simulation. However, for certain pressures (for example, 8 GPa) this hysteresis becomes minuscule, and the cooling/heating curves nearly overlap. When the area A H ( A V ) of the enthalpy (volume) hysteresis is followed as a function of pressure ( Fig. 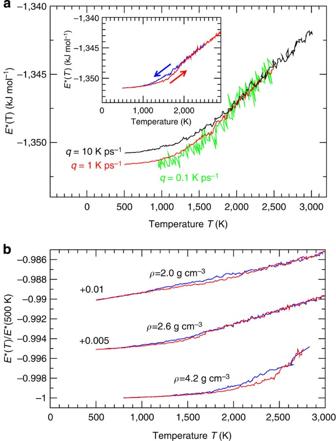3b ), a deep minimum is found, indicating that glasses in that pressure range must display a quite different relaxation behaviour that leads to a RW. Figure 2: A numerical glass transition cycle. (a) Evolution in (N,V,T) ensemble (ρ=3.2 g cm−3) of the liquid potential energyE*(T) with temperature for different cooling rates. All are represented after subtraction of 9RT/2 to account for the harmonic motions in the glassy state upon cooling. The inset shows a typical cooling/heating cycle (q=1 K ps−1) for the same system. (b) Evolution in (N,V,T) ensemble of the liquid potential energyE*(T) with temperature during a cooling (blue) and heating (red) cycle (1 K ps−1) for different system densities. All are represented after subtraction of 9RT/2 to account for the harmonic motions in the glassy state, and rescaled with respect to the valueE*(500 K). Figure 2: A numerical glass transition cycle. ( a ) Evolution in ( N , V , T ) ensemble ( ρ =3.2 g cm −3 ) of the liquid potential energy E* ( T ) with temperature for different cooling rates. All are represented after subtraction of 9 RT /2 to account for the harmonic motions in the glassy state upon cooling. The inset shows a typical cooling/heating cycle ( q =1 K ps −1 ) for the same system. ( b ) Evolution in ( N , V , T ) ensemble of the liquid potential energy E* ( T ) with temperature during a cooling (blue) and heating (red) cycle (1 K ps −1 ) for different system densities. All are represented after subtraction of 9 RT /2 to account for the harmonic motions in the glassy state, and rescaled with respect to the value E* (500 K). Full size image Figure 3: Effect of pressure on the cooling/heating cycle across the glass transition. ( a ) Volume-temperature dependence in ( N , P , T ) ensemble during a cooling (red) and heating (blue) cycle for selected pressures of liquid 2SiO 2 –Na 2 O across the glass transition. The volumes have been rescaled with respect to their evolution in the glassy state V glass ( T ). Curves at 0 and 8 GPa have been shifted by multiples of 0.1. The cycle leads to a hysteresis, which is due to structural relaxation. ( b ) Area of the enthalpic ( A H ) and volumetric ( A V , red curve, right axis) hysteresis as a function of the applied pressure P , defining a reversibility window (RW, grey zone). Full size image Relationship with structure To investigate the relationship between the anomalous relaxation dynamics highlighted in Fig. 3 , and structural properties, we first represent in Fig. 4a the calculated fraction of n -fold coordinated silicon species ( n =4, 5, 6) as a function of pressure in the vicinity of the glass transition. Coordination change in silica and silicates are well documented both experimentally [11] and by computer simulations [12] , [13] , [14] , and indicate the usual transformation of tetrahedral order ( n =4), which prevails at ambient conditions, into octahedral order ( n =6) that dominates at elevated pressure. Here we find indeed that the four-fold tetrahedral Si progressively converts into an intermediate coordination ( n =5), whereas the higher coordinated Si ( n =6) increases only for pressures larger than 20 GPa, consistently with the most recent MD simulations of a similar system (silica) that have been validated by in situ high-pressure diffraction experiments [14] . These trends obviously do not provide any direct correlation with the obtained anomaly in volume and enthalpy recovery. 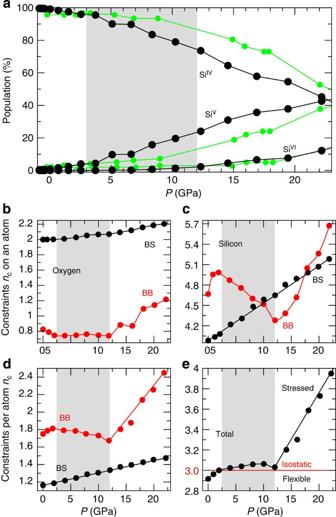Figure 4: Structure and constraint behaviour of densified silicates. (a) Behaviour of then-fold coordinated Si (black) species in liquid 2SiO2–Na2O as a function of pressure (2,000 K), compared with recent results for simulated amorphous silica (green14). The grey zone corresponds to the approximate boundaries of the RW window ofFig. 2b. (b) Calculated number of bridging oxygen stretching- and bending constraintsncBS(BO) andncBB(BO) as a function of pressure. (c) Calculated number of Silicon stretching- and bending constraintsncBS(Si) andncBB(Si). (d) Corresponding total bond-stretchingncBSand bond-bending constraints per atomncBB. (e) Total number of constraints per atom of the NS2 system. The horizontal red line represents the isostatic linenc=3 (Maxwell stability criterion), and separates flexible from stressed rigid networks. Figure 4: Structure and constraint behaviour of densified silicates. ( a ) Behaviour of the n -fold coordinated Si (black) species in liquid 2SiO 2 –Na 2 O as a function of pressure (2,000 K), compared with recent results for simulated amorphous silica (green [14] ). The grey zone corresponds to the approximate boundaries of the RW window of Fig. 2b . ( b ) Calculated number of bridging oxygen stretching- and bending constraints n c BS (BO) and n c BB (BO) as a function of pressure. ( c ) Calculated number of Silicon stretching- and bending constraints n c BS (Si) and n c BB (Si). ( d ) Corresponding total bond-stretching n c BS and bond-bending constraints per atom n c BB . ( e ) Total number of constraints per atom of the NS2 system. The horizontal red line represents the isostatic line n c =3 (Maxwell stability criterion), and separates flexible from stressed rigid networks. Full size image Topological constraints and evidence for adaptation Next, we introduce a measure of stress in the liquid ( Fig. 4b–d ) by computing parameters that quantify the radial and angular excursions between pairs or triplet of atoms. This is directly inspired by the classical mechanics view of topological constraints associating large/small radial or angular motion with the absence/presence of corresponding bond-stretching (BS) and bond-bending (BB) restoring forces [15] , [16] . By building on the concept of Maxwell rigidity [5] , [6] , earlier work on amorphous networks [17] , [18] has shown that such BS constraints can actually be simply enumerated from the coordination number r i of the atoms, leading to a contributions of r i /2 for the BS constraint, each bond/interaction being shared by two neighbours. Given the increase of the Si and O coordination with pressure ( Fig. 4a ), one thus automatically acknowledges an increase in the corresponding BS constraints n c BS (black curves, Fig. 4b,c ). To derive angular (BB) constraints, we follow the angular motion around each individual atom k ( k =O, Si) defined by a set of two neighbours. Over the time MD trajectory, the corresponding bond-angle distribution P k ( θ ) allows defining a mean (the first moment of P k ( θ )) and a standard deviation σ k (the second moment) that shows a bimodal distribution f ( σ k ) for various thermodynamic conditions [15] , [19] . Atoms subject to a rigid bending interaction contribute to the part of f ( σ k ) with low σ k (typically, σ k <10°), have a corresponding angle that acts as a rigid BB constraint, and induce network stiffening. Averages over the whole system then lead to the mean number of constraints n c BB per atom. Figure 4b,c shows the calculated evolution of the number of BB constraints n c BB of the oxygen and silicon as a function of pressure (red curves). Starting from 0 GPa, n c BB (Si) increases with pressure, whereas n c BB (O) decreases, and for the total system ( Fig. 4d ), the number of BB constraints per atom increases given that the evolution is mostly triggered by the 6 angles defining the Si tetrahedra. However, at a pressure of about 3 GPa, the system attains an obvious threshold. Further compression now leads to a decrease of n c BB (Si), and to a global decrease of n c BB ( Fig. 4d ), and this evolution holds up to a pressure of about 12 GPa beyond which an important growth of all constraints takes place. Taken together, the results ( Fig. 4d ) indicate an obvious correlation between these determined threshold pressures and those obtained for thermal quantities during the cooling/heating cycle ( Fig. 3 ). While the change in structure itself may not affect directly the properties during the cycle ( Fig. 4a ), it becomes clear from the location of the obtained thresholds that the way the interactions (or constraints) behave with pressure influences the dynamics (see below) during the glass transition that ultimately affects the shape of the hysteresis. Finally, the total number of constraints for the system shows a plateau-like behaviour ( Fig. 4e ) at a value n c =3 between ~3 and 12 GPa, which, again, can be put in parallel with the evolution of the hysteresis areas A V and A H , displayed in Fig. 3b . Relaxation and dynamic behaviour For the present simulations of densified silicates, when the viscosity η is calculated (Green–Kubo [8] ) and followed with inverse temperature in an Arrhenius plot ( Fig. 5a ), a linear behaviour is obtained, that is, η behaves as η = η 0 exp[ E A / k B T ]. The corresponding activation energies E A display a similar minimum with pressure [9] , and when represented as a function of the calculated number of constraints, it is found that the minimum in E A coincides with n c =3 (top inset of Fig. 5a ). In addition, the relaxation time τ at T =2,000 K is found to evolve similarly. Here one assumes the Maxwell relation η=G ∞ τ with G ∞ the instantaneous shear modulus, and a separate computation of the viscosity η , and G ∞ from the shear strain/shear stress response [20] provides the evolution of τ with respect to pressure P or constraint density n c . A deep minimum is found in the relaxation time ( τ ~2–3 ps) in the region 3.0< n c <3.2 (bottom inset of Fig. 5a ), leading, again, to an appealing anomaly. 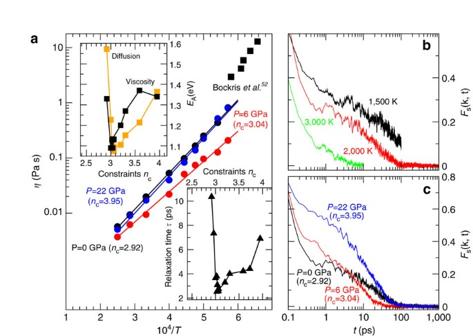Figure 5: Calculated dynamic quantities of NS2 as a function of pressure and temperature. (a) Arrhenius plot of the Green–Kubo-calculated viscosities for selected pressures and indicated number of constraints (2.92, 3.04 and 3.95) per atom at 2,000 K. The data at 0 GPa (nc=2.92) can be compared with experimental values of viscosity (Bockriset al.53) measured at ambient conditions. The top inset shows the corresponding activation energyEA(black symbols), together with corresponding calculated activation energy for diffusionEA(orange symbols), derived from an Arrhenius plot of oxygen diffusivity54. The bottom inset shows a calculated relaxation timeτas a function ofncdetermined from a separate evaluation of the viscosity and the instantaneous shear modulus20. (b) Oxygen intermediate scattering functionFs(k,t) of aP=0 NS2 liquid atk=kmax=3.04 A−1for different temperatures. Note thatkmaxcorresponds to the principal peak position of the static structure factorS(k), and remains nearly constant with thermodynamic conditions9. (c) Oxygen intermediate scattering functionFs(kmax,t) atT=2,000 K for different constraints/pressures. Figure 5: Calculated dynamic quantities of NS2 as a function of pressure and temperature. ( a ) Arrhenius plot of the Green–Kubo-calculated viscosities for selected pressures and indicated number of constraints (2.92, 3.04 and 3.95) per atom at 2,000 K. The data at 0 GPa ( n c =2.92) can be compared with experimental values of viscosity (Bockris et al . [53] ) measured at ambient conditions. The top inset shows the corresponding activation energy E A (black symbols), together with corresponding calculated activation energy for diffusion E A (orange symbols), derived from an Arrhenius plot of oxygen diffusivity [54] . The bottom inset shows a calculated relaxation time τ as a function of n c determined from a separate evaluation of the viscosity and the instantaneous shear modulus [20] . ( b ) Oxygen intermediate scattering function F s ( k , t ) of a P =0 NS2 liquid at k=k max =3.04 A −1 for different temperatures. Note that k max corresponds to the principal peak position of the static structure factor S ( k ), and remains nearly constant with thermodynamic conditions [9] . ( c ) Oxygen intermediate scattering function F s ( k max , t ) at T =2,000 K for different constraints/pressures. Full size image To track the effect of pressure on the dynamic and relaxation behaviour of the supercooled NS2 liquid, we finally compute the intermediate scattering function F s ( k , t ). This function follows the Fourier components of density correlations, and characterizes the slowing down of the relaxation that can be investigated for different temperatures and different pressures, for example, at wavectors k=k max , the principal peak position of the static structure factor S ( k ). Here, F s (k, t ) exhibits at the lowest considered temperature (1,500 K) the usual two-step relaxation behaviour with a plateau (for example, at F s ( k , t )~0.3 for T =1,500 K, Fig. 5b ) that is similar to the case of silica [21] . This behaviour builds up as the temperature is decreased, consistently with the loss of a single-step relaxation behaviour that is typical of high-temperature liquids (3,000 K). The same dynamic behaviour can be investigated along an isotherm (2,000 K, Fig. 5c ) as a function of pressure, to establish a link with the adaptive regime obtained from the topological analysis ( Fig. 4 ), and is discussed below. The value n c =3 per atom ( Fig. 4e ) actually has a deeper meaning. It corresponds to the well-known Maxwell stability criterion [5] , [6] of isostatic structures [17] , and has been identified in glasses as the location of a mean-field rigidity transition [17] , [18] , which separates flexible or underconstrained glasses ( n c <3, with low-frequency (floppy) deformation modes involving energies of about 5 meV [22] ) from overconstrained networks ( n c >3) in which stressed rigidity dominates. Having obtained all separated evolutions of n c BS and n c BB , we now realize that with the pressure-imposed coordination change leading to a growth of network connectivity and stretching interactions ( n c BS ), the energetically weaker interactions (BB) [22] soften to accommodate the increase of stress. The angular adaptation reducing n c BB (as sketched in Fig. 6 ) preserves a stress-free state and the isostatic nature ( n c =3) of the network backbone over a finite pressure interval. However, this adaptive situation holds only up to a certain point given that both Si and O coordination numbers ( Fig. 4a ), and stress induced by stretching interactions will continue to increase with pressure. The limit is obviously found at 12 GPa where angles stiffen and BB constraints are restored. The total number of constraints n c then grows substantially with pressure. Remarkably, the plateau behaviour n c ~3 ( Fig. 4e ) is found where thermal reversibility and volumetric recovery are obtained, and these windows are essentially driven by the adaptation of the angles. 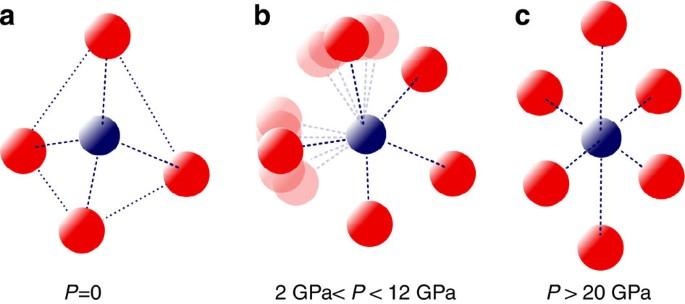Figure 6: A schematic representation of angular adaptation. Typical local structures in densified 2SiO2–Na2O supercooled liquids and glasses: (a) a SiO4/2tetrahedron (dominant atP=0, and in α-quartz10), (b) a fivefold coordination Si (n=5) whose population grows as pressure increases (see, for example, ref.14) and (c) an octahedral (n=6) Si, the dominant motif at elevated pressures (P>20 GPa) and in the crystalline stishovite polymorph10. In the reversibility windows (RW), the angular excursion (O–Si–O) increases (Fig. 3c) to accommodate stress, and leads to a softening of the bending interaction (b). This preserves the isostatic character of the network over a finite pressure interval. Figure 6: A schematic representation of angular adaptation. Typical local structures in densified 2SiO 2 –Na 2 O supercooled liquids and glasses: ( a ) a SiO 4/2 tetrahedron (dominant at P= 0, and in α-quartz [10] ), ( b ) a fivefold coordination Si ( n= 5) whose population grows as pressure increases (see, for example, ref. 14 ) and ( c ) an octahedral ( n= 6) Si, the dominant motif at elevated pressures ( P >20 GPa) and in the crystalline stishovite polymorph [10] . In the reversibility windows (RW), the angular excursion (O–Si–O) increases ( Fig. 3c ) to accommodate stress, and leads to a softening of the bending interaction ( b ). This preserves the isostatic character of the network over a finite pressure interval. Full size image We are not aware of any experimental work showing reversibility driven by pressure in glass-forming liquids. However, in rigidity transitions driven by chemical alloying, experimental calorimetric RWs (Boolchand phases) have been reported such as in Ge x Se 1− x glasses [23] . For the latter, the increase of stress is achieved by the addition of Ge crosslinks into the flexible Se-rich network structure. At some point in the compositional space, simple lattice models indicate that stress induced by such crosslinks can be accommodated and partially released during the glass transition because stress-free sub-regions percolate, and are able to maintain a nearly isostatic character over a finite interval in composition [24] , [25] . A large number of experimentally investigated chalcogenide, modified oxides and heavy-metal-oxide glasses exhibits a RW ( Fig. 7 ). We represent, among other systems, very different glasses with ionic, iono-covalent, covalent or semi-metallic character such as Ge–X (X=S, Se (refs 23 , 26 )), Ge–S–I (ref. 27 ), AgPO 3 –AgI (ref. 28 ), Ge–Te–In–Ag (ref. 29 ), SiO 2 –Na 2 O (ref. 30 ) or TeO 2 –V 2 O 5 (ref. 31 ). 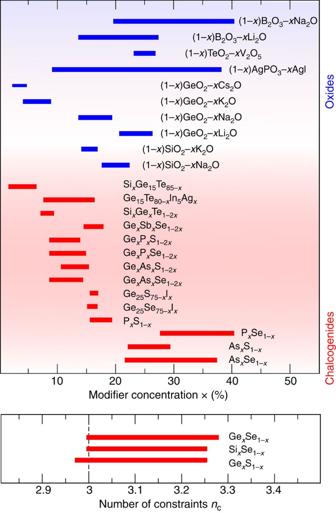Figure 7: Location of experimental reversibility windows (Boolchand phases). (a,b) Si–Se (ref.32), Ge–Se (ref.23), Ge–S (ref.26), As–Se (ref.55), As–S (ref.36), P–Se (ref.56), P–S (ref.33), Ge–Se–I (ref.34), Ge–S–I (ref.27), Ge–As–Se (ref.35), Ge–As–S (ref.37), Ge–P–Se (ref.45), Ge–P–S (ref.57), Ge–Sb–Se (ref.58), Si–Ge–Te (refs59,60) Ge–Te–In–Ag (ref.29), SiO2–M2O (M=Na, K) (ref.30), GeO2–M2O (M=Li, K, Cs) (P. Boolchand, unpublished results), GeO2–Na2O (ref.61), AgPO3–AgI (ref.28), TeO2–V2O5(ref.31) and B2O3–M2O (M=Li, Na) (ref.62). Note the effect of the cation size in the same families of modified oxides. (b) Using the 8−N(octet) rule, the RW can be represented only for a very limited number of systems as a function of the number of mechanical constraints (panel b) using the mean-field estimate ofnc17,18, and is found close tonc=3. Figure 7: Location of experimental reversibility windows (Boolchand phases). ( a , b ) Si–Se (ref. 32 ), Ge–Se (ref. 23 ), Ge–S (ref. 26 ), As–Se (ref. 55 ), As–S (ref. 36 ), P–Se (ref. 56 ), P–S (ref. 33 ), Ge–Se–I (ref. 34 ), Ge–S–I (ref. 27 ), Ge–As–Se (ref. 35 ), Ge–As–S (ref. 37 ), Ge–P–Se (ref. 45 ), Ge–P–S (ref. 57 ), Ge–Sb–Se (ref. 58 ), Si–Ge–Te (refs 59 , 60 ) Ge–Te–In–Ag (ref. 29 ), SiO 2 –M 2 O (M=Na, K) (ref. 30 ), GeO 2 –M 2 O (M=Li, K, Cs) (P. Boolchand, unpublished results), GeO 2 –Na 2 O (ref. 61 ), AgPO 3 –AgI (ref. 28 ), TeO 2 –V 2 O 5 (ref. 31 ) and B 2 O 3 –M 2 O (M=Li, Na) (ref. 62 ). Note the effect of the cation size in the same families of modified oxides. ( b ) Using the 8− N (octet) rule, the RW can be represented only for a very limited number of systems as a function of the number of mechanical constraints (panel b) using the mean-field estimate of n c [17] , [18] , and is found close to n c =3. Full size image For the simplest systems, that is, binary network glasses such as Si x Se 1− x or Ge x S 1− x , the experimental boundaries of the RW are found to be all very close, that is, roughly located between x =20% and x =25% ( Fig. 7b ). A direct relationship can then be made with the isostatic nature of the network given the well-defined coordination numbers of Ge/Si and S/Se that follow the 8- N (octet) rule ( N being the number of s and p electrons). For such glasses, the lower boundary of the RW (for example, x =20% Ge in Ge–Se) is, indeed, found to coincide with the Phillips–Thorpe [17] , [18] mean-field constraint count n c =3. Aspects of topology here fully control the evolution of rigidity with increasing group IV content, and there is a weak chemical effect due to Ge/Si or S/Se substitution [23] , [26] , [32] . For most of the systems, however, coordination numbers and related active/inactive constraints must be derived from specific structural models [27] , [33] , [34] , [35] . This becomes already obvious when isochemical glasses (group V selenides/sulphides) are considered ( Fig. 7a ), because different RW locations emerge between sulphides and selenides, and between As- and P-bearing chalcogenides. The validity of these structural models is still debated in the literature, although rather well established in some cases from spectroscopic studies [33] , [36] , [37] . These conclusions can be maintained to some extent for the wide class of modified oxides ( Fig. 7a ), which display the same phenomenology as the chalcogenide networks, that is, a RW is found between the two end limits of possible networks or elastic phases. These networks/phases can be either highly connected and stressed rigid (for example, silica-rich silicates), or strongly depolymerized and flexible (for example, pyrosilicates SiO 2 –2Na 2 O) [30] . The physical picture that emerges from our findings is the following. In densified NS2 liquids, the RW is a direct consequence of the formation of an isostatic structure that minimizes both stress ( n c >3) and the low-frequency deformation (floppy, n c <3), a direct consequence of two opposite trends with pressure. Without stress (present at low pressures) that induces bond/stress relaxation and without floppy modes (present at high pressures) that lead to low-energy relaxation phenomena, an adaptive isostatic system will lead to significantly reduced relaxation times that minimizes the enthalpic overshoot and the hysteresis appearing in the glass transition cycles. A first support for this idea has been given from a modified Debye model [38] describing in a simple way the effect of rigidity on the relaxation in relationship with the underlying energy landscape [2] . The roughness of the landscape is then determined by both the bond and the floppy mode density, the former (an increasing function of pressure or connectivity) contributing to energy basins or inherent structures, while the latter (a decreasing function of pressure) leads to channels in the landscape, which extend the possibilities of relaxation. A second simple result supporting our view arises from a Keating model reproducing both floppy modes and BS and BB interactions (stress) [39] . By following a Metropolis algorithm in a Monte Carlo approach of the glass transition, it has been found that isostatic systems have a higher acceptation rate for energy changes, and this leads to an enhanced relaxation at low temperature that manifests also by a minimum in the activation energy E A of the relaxation time τ=τ 0 exp( E A /k B T ). An inspection of Fig. 4a (minimum in E A , minimum in τ ) shows that the conclusions derived from these simple models [38] , [39] are recovered for the present simulated NS2 liquids. Results from Fig. 5a indicate, indeed, that the energy barriers for viscous relaxation are lower, and that the evolution of the viscosity with inverse temperature is smaller for pressures belonging to the RW. With a slower temperature evolution of the relaxation time for isostatic systems close to the glass transition, faster changes in energy are expected to occur with the imposed cooling/heating rate, and will result in a cycle with a reduced area for the relaxation time τ , which minimize for isostatic glass-forming liquids (bottom inset of Fig. 5a ). The second piece of evidence for anomalous dynamic behaviour that leads to reversibility for isostatic systems is provided by the calculated intermediate scattering function F s ( k , t ) ( Fig. 5b,c ). When represented along a select isotherm ( T =2,000 K) for different pressures ( Fig. 5c ), it is found that pressure does not affect the time evolution of the different intermediate scattering functions F s ( k , t ) in a monotonic fashion. In the microscopic regime at low times ( t <1 ps), flexible liquids (low-pressurized NS2) relax more rapidly given that floppy modes are present that facilitate relaxation on the local scale involving short times typical of a high-temperature liquid. Furthermore, for such liquids, small but visible oscillations at around t ~0.5–0.8 ps are found ( Fig. 5b and black curve Fig. 5c ), corresponding to frequencies of about 1.25–2 THz (5–8 meV), that is, to frequencies that are typical of floppy modes [22] . These features are virtually absent in isostatic and stressed rigid systems, or are, at least, substantially reduced. For longer times ( t >5 ps) typical of α-relaxation timescales [21] ( β -relaxation being barely observed in Fig. 5c at the considered temperature), it is seen that isostatic glasses now relax faster as also noticed from the calculated relaxation time from viscosity (bottom inset, Fig. 5a ). These systems relax, indeed, to F s ( k , t )=0 at timescales (20 ps) that are 4–5 times smaller than those of flexible or stressed glass-forming liquids, this statement remaining valid for different wavenumbers (not shown). It indicates the very special nature of systems fulfilling n c =3, and this enhanced ease to α-relaxation obtained from various dynamic probes is, obviously, correlated to the thermodynamic results and anomalies appearing in the glass transition cycle. A certain number of broader consequences can be sketched. First, the present results connect to the notion of glass-forming ability, that is, the ease to from glasses from the liquid state, and the associated thermal stability with respect to recrystallization at T=T x , once a liquid has been quenched to a glass. Crystallization can be hardly achieved on computer timescales (see however ref. 40 ) so that a direct connection between isostaticity and thermal stability cannot be made for the present densified silicates. However, experiments reveal that glass stability, quantified by the quantity Δ T=T x −T g , is enhanced for such isostatic compositions. In RWs obtained by changes in composition, Δ T is, indeed, found to be maximum, indicating an increased thermal stability [29] , [41] . Similarly, select compositional studies on silicates show that a minimum in the critical cooling rate to avoid crystallization [42] coincides with the location of the RW [30] . A natural question that emerges at this stage is the degree of generality of the established relationship between adaptive isostaticity and reversibility. Does this relationship apply to all glasses? Here, we have focused on an ionic system constrained only by directional bond and angular interactions, and reviewed ionic, iono-covalent and covalent glasses exhibiting experimental RWs. Results appear to be generic because the same experimental behaviour is reported for a variety of glass systems, simple chalcogenides, ternary compounds, binary oxide glasses, chalcohalides, heavy metal oxides and so on, and these bear striking similarities with the pressure-driven RW determined from the MD simulations. An extension to, for example, metallic glasses involving non-directional interactions, or to other types of disordered systems for which glassy behaviour can be achieved, would require a neat definition of the forces constraining the system. Recent work [43] on hard-sphere systems constrained only by contact forces has shown that the salient features of mean-field rigidity [17] , [18] could be recovered from a vibrational analysis. This represents an interesting starting result for future investigations of possible reversibility and RWs [44] of hard spheres glass-forming liquids. The realization of stress-free networks, and the detection of glasses having a reversible character where relaxation is obviously minimized, and accompanied by other anomalous behaviours, may be used for the design of materials with specific applications. It has indeed been found experimentally that stress-free glasses display weak ageing phenomena and thermal stability [29] , [41] , [45] , while also having a reduced plastic behaviour [46] . The present result also connects to the field of ‘Topological Engineering’, which has recently emerged in materials science [47] , and which enables the design of new functionalities using as simple inputs the topology and the rigidity of the underlying molecular network. Promising applications have been reported in this context. Gorilla Glass [48] serves as a protective sheet in cell phones, and its hardness (a very crucial parameter regarding cell phone lifetime) [49] and process parameters (viscosity and glass transition temperature) can be optimized from an atomic-scale approach using the topological constraint density and the isostatic criterion [47] , [49] . Cement [50] and concrete properties are known to heavily depend on the C–S–H ratio between CaO, SiO 2 and H 2 O. An application of rigidity and constraint-counting algorithms [51] have shown that cement with a CaO/SiO 2 ratio of 1.5 is isostatic, this composition defining two broad categories of materials with different mechanical responses (strong transverse versus isotropic), while also exhibiting an indentation modulus-to-hardness ratio maximum. Finally, the anomalous relaxation phenomena that are revealed by RWs and detailed atomic-scale simulations may be used for the design of innovative semiconductors having a reduced capacitive power loss [52] . Here connectivity and rigidity of the relevant materials are tuned by hydrogenating Si–C alloys, and subsequently roughly analysed from a mean-field constraint count [17] , [18] . At present, issues related to reversibility, thermal stability and adaptability of the underlying atomic-scale networks have not been considered so far in such semiconducting alloys, but it is quite remarkable and unexpected that such dissimilar modern applications, glasses, cement and semiconducting alloys, can all be traced back to Maxwell’s stability criterion using the notion of isostaticity. Molecular Dynamics simulations The system under investigation is composed of 3,000 atoms that interact via a Born–Mayer pair-wise potential (J. Teter, unpublished results), which has been found to accurately reproduce experimental data on structure and dynamics [7] , [8] , [9] . Simulations have been performed both in ( N , V , T ) with 1.6 g cm −3 < ρ <4.2 g cm −3 (for example, Fig. 2a ) and ( N , P , T ) ensemble with 0< P <22 GPa to check for consistency. After equilibrating the systems at 3,000 K for 1 ns, a linear cooling/heating ramp has been applied under various isochoric or isobaric conditions, down to 300–500 K. Several different initial configurations have been used in three independent quenches. During the heating simulations, both enthalpy and volume (in N , P , T ) or energy (in N , V , T ) exhibited a hysteresis ( Fig. 2b ), and the area of this hysteresis has been tracked as a function of thermodynamic conditions (pressure P or volume V ). How to cite this article: Bauchy, M. et al . Densified network glasses and liquids with thermodynamically reversible and structurally adaptive behaviour. Nat. Commun . 6:6398 doi: 10.1038/ncomms7398 (2015).